Intracellular chloride concentration influences the GABAAreceptor subunit composition GABA A receptors (GABA A Rs) exist as different subtype variants showing unique functional properties and defined spatio-temporal expression pattern. The molecular mechanisms underlying the developmental expression of different GABA A R are largely unknown. The intracellular concentration of chloride ([Cl − ] i ), the main ion permeating through GABA A Rs, also undergoes considerable changes during maturation, being higher at early neuronal stages with respect to adult neurons. Here we investigate the possibility that [Cl − ] i could modulate the sequential expression of specific GABA A Rs subtypes in primary cerebellar neurons. We show that [Cl − ] i regulates the expression of α3-1 and δ-containing GABA A receptors, responsible for phasic and tonic inhibition, respectively. Our findings highlight the role of [Cl − ] i in tuning the strength of GABAergic responses by acting as an intracellular messenger. The GABAergic system undergoes profound developmental changes. Most remarkably, during development, GABA A action shifts from depolarizing to hyperpolarizing [1] . The polarity of GABA responses depends upon the intracellular chloride concentration ([Cl − ] i ), which is mainly controlled by the action of Na + -K + -2Cl − (NKCC1) and K + -Cl − (KCC2) co-transporters. In the immature brain, NKCC1 expression determines high [Cl − ] i , promoting depolarizing GABA responses which has been demonstrated to lead to excitation by promoting sodium action potential triggering, voltage-gated calcium channel activation and generation of giant depolarizing potentials [2] , [3] . In addition, depolarizing GABA action can also lead to inhibition due to the presence of shunting inhibition that, in turn, critically depends on the chloride driving force and the synapse location [4] , [5] . In contrast, in the adult brain, chloride extrusion operated by KCC2 establishes low [Cl − ] i, with consequent inhibitory action of GABA A ergic currents. Such developmental chloride gradient inversion is assumed to occur in all neurons of the central nervous system (CNS), although its timing can significantly vary in various brain regions and neuronal subtypes [1] , [6] , [7] . In addition to the [Cl − ] i changes, the expression of distinct post-synaptic GABA A receptor (GABA A R) subtypes also undergoes developmental regulation [8] . In the cerebellum, immature GABAergic synapses express α3-containing GABA A R that are progressively replaced by α1-containing receptors at mature synapses [9] , [10] . Such GABA A R-subtype switch underlies the developmental speed-up from the slow decay kinetics of α3-containing GABA A Rs to the fast decay kinetics of α1-containing GABA A Rs [9] , [10] , [11] . It is believed that long-lasting α3-mediated currents promote trophic actions in immature neurons, whereas fast α1-mediated hyperpolarizing spontaneous inhibitory postsynaptic currents (sIPSCs) contribute to increase the network temporal resolution in mature neurons [9] , [10] , [12] . Moreover, tonic current has been shown to increase over development in cerebellar acute slices due to the progressive expression of the δ subunit [10] , [13] . The molecular mechanisms underlying the developmental α3 to α1 switch and δ subunit up-regulation are poorly understood. Since the shift in the polarity of chloride gradient occurs in parallel with the α3 to α1 GABA A R subunit switch during the first two postnatal weeks, in this study we investigated whether changes in [Cl − ] i interfere with the surface expression of α3 and α1 subunits by using a genetic and pharmacological approach. Electrophysiological and immunocytochemistry results demonstrated that the intracellular chloride concentration regulates the expression of α3-α1 and δ subunits of GABA A Rs, thereby influencing both the kinetics of sIPSCs and the amount of tonic inhibition. α3-1 and δ subunits are affected by KCC2 or Bumetanide To investigate the role of [Cl − ] i in the regulation of α and δ subunit expression of GABA A Rs, we studied the decay kinetics of spontaneous GABA A ergic currents and the expression of α3/α1 subunits in cerebellar neurons (stellate/basket cells, Methods). To this end, in a first set of experiments, the [Cl − ] i was reduced by over-expression of KCC2 in immature neurons on the day of the plating ( Fig. 1a ). As expected, gramicidin perforated patch-clamp experiments revealed that, in cultures at days in vitro 6–7 (DIV6–7), the reduced [Cl − ] i resulting from KCC2 over-expression reverted GABA A current polarity from depolarizing to hyperpolarizing responses ( E Cl : −38±4 and −64±7 mV in control and KCC2 over-expression, respectively, P <0.01 unpaired t -test, V m: 55.0±3.4 mV; Fig. 2a–c ). Notably, these data were corroborated by immunocytochemistry showing an increased KCC2 immunoreactivity in KCC2 over-expressing neurons at DIV6–7 ( Fig. 2d,e ). The GABAergic sIPSCs from DIV6–7 was recorded under over-expression of KCC2. Interestingly, KCC2 over-expression accelerated the relaxation of sIPSCs, leaving unchanged their frequency ( Fig. 2f–h ) and did not affect the density of GABAergic synapses as confirmed by VGAT immunostaining ( Fig. 2i,j ). Since the GABA A R-mediated tonic current is also developmentally regulated in acute slices, being small in immature neurons and progressively larger during development [10] , [13] , we investigated whether it was also affected in KCC2 over-expressing neurons. As shown in Fig. 2k , DIV6–7 neurons over-expressing KCC2 displayed larger tonic current amplitude than untreated neurons. This set of data supports the hypothesis that over-expression of KCC2 might influence the expression of α3/α1 and δ GABA A R subunits, crucial for both the kinetics of synaptic currents and the amplitude of tonic GABA current, respectively. To further demonstrate this hypothesis, the relative amount of GABA A R α3, α1 and δ subunits in neurons with low [Cl − ] i was studied by immunocytochemistry. As shown in Fig. 2l,m KCC2 over-expression in DIV6–7 neurons led to an increase in the expression of α1 subunit, whereas the α3 subunit was expressed to a lower extent in comparison to controls. In a second set of immunocytochemistry experiments, we observed that the surface expression of δ subunit was also increased in KCC2 over-expressing neurons at DIV 6–7 ( Fig. 2n,o ). Taken together, these data corroborate the electrophysiological results, and suggest that the developmental expression of GABA A R α3−α1 and δ subunits is regulated by KCC2 expression. 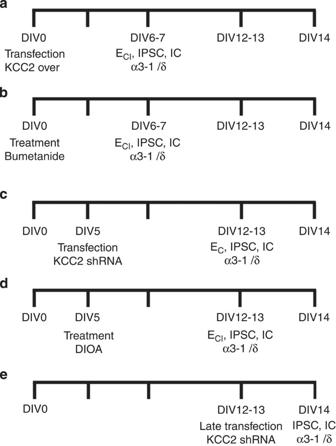Figure 1: Summary of experimental procedures timing for the genetic and pharmacological approches. (a) In KCC2 over-expression experiments, transfection was performed at DIV0 whereas the recordings of IPSCs,EClmeasurements and immunocytochemistry (IC) were performed at DIV 6–7. (b) In chronic Bumetanide experiments, the drug was applied at DIV0 whereas the recordings of IPSCs,EClmeasurements and immunocytochemistry (IC) were performed at DIV 6–7. (c) In KCC2 shRNA experiments, transfection was performed at DIV5 whereas the recordings of IPSCs,EClmeasurements and immunocytochemistry (IC) were performed at DIV12–13. (d) In chronic DIOA experiments, the drug was applied at DIV5 whereas the recordings of IPSCs,EClmeasurements and immunocytochemistry (IC) were performed at DIV 12–13. (e) In late transfection of KCC2 shRNA experiments, trasfection was performed at DIV12–13 whereas the recordings of IPSCs and immunocytochemistry (IC) were performed at DIV14. Figure 1: Summary of experimental procedures timing for the genetic and pharmacological approches. ( a ) In KCC2 over-expression experiments, transfection was performed at DIV0 whereas the recordings of IPSCs, E Cl measurements and immunocytochemistry (IC) were performed at DIV 6–7. ( b ) In chronic Bumetanide experiments, the drug was applied at DIV0 whereas the recordings of IPSCs, E Cl measurements and immunocytochemistry (IC) were performed at DIV 6–7. ( c ) In KCC2 shRNA experiments, transfection was performed at DIV5 whereas the recordings of IPSCs, E Cl measurements and immunocytochemistry (IC) were performed at DIV12–13. ( d ) In chronic DIOA experiments, the drug was applied at DIV5 whereas the recordings of IPSCs, E Cl measurements and immunocytochemistry (IC) were performed at DIV 12–13. ( e ) In late transfection of KCC2 shRNA experiments, trasfection was performed at DIV12–13 whereas the recordings of IPSCs and immunocytochemistry (IC) were performed at DIV14. 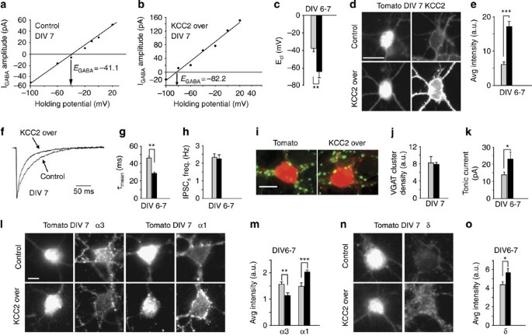Figure 2: KCC2 over-expression affects GABAergic currents and regulates the expression of α3-α1 and δ subunits. (a) Example ofI–Vrelations of isoguvacine (10 μM) evoked GABAAcurrents at increasing holding potentials in control neurons. (b) Example ofI–Vrelations of isoguvacine (10 μM) evoked GABAAcurrents at increasing holding potentials in KCC2 over-expressing neurons. (c) Bar plot showing the meanEClin immature neurons (control, grey barn=6; KCC2 over, black barn=7; **P<0.01; unpairedt-test). (d) Somatic KCC2 immunostaining in control and KCC2 over-expressing neuron. (Scale bar: 5 μm). (e) Quantification of KCC2 immunofluorescence signals in control and KCC2 transfected neurons (control, grey barn=16; KCC2 over, black barn=20; ***P<0.001; unpairedt-test). (f) Representative sIPSCs from control and KCC2 transfected neurons. (g) Summary of sIPSC decay kinetics in control (grey barn=44) and KCC2 transfected neurons (black barn=37; **P<0.01; unpairedt-test). (h) Summary of sIPSC frequency in control (grey barn=41) and KCC2 transfected neurons (black barn=40;P>0.05; unpairedt-test). (i) Immunostaining of VGAT clusters (green fluorescence) in control (left panel) and KCC2 over-expressing neurons (right panel). (j) Summary of VGAT cluster density quantification in control (grey barn=19) and KCC2 transfected neurons (black barn=24;P>0.05; unpairedt-test). (k) Summary of tonic current amplitude in control (grey barn=43) and KCC2 neurons (black barn=28; *P<0.05; unpairedt-test). (l) Somatic immunostaining of immunofluorescence signals for α3 and α1 subunits in control and KCC2 over-expressed neurons at DIV7, scale bar 10 μm. (m) Quantification of immunofluorescence signals for α3 and α1 subunits at DIV7 (α3 control, grey barn=69; KCC2 over, black barn=75; **P<0.01; unpairedt-test; α1 control grey barn=104; KCC2 over black barn=121; ***P<0.001; unpairedt-test). (n) Somatic immunostaining of immunofluorescence signals for δ subunit in control and KCC2 over-expressing neurons at DIV7. (o) Quantification of immunofluorescence signals for δ subunit (control, grey barn=17; KCC2 over, black barn=42; *P<0.05; unpairedt-test). Scale bar: 23 μm. Data is presented as mean±s.e.m. Full size image Figure 2: KCC2 over-expression affects GABAergic currents and regulates the expression of α3-α1 and δ subunits. ( a ) Example of I – V relations of isoguvacine (10 μM) evoked GABA A currents at increasing holding potentials in control neurons. ( b ) Example of I – V relations of isoguvacine (10 μM) evoked GABA A currents at increasing holding potentials in KCC2 over-expressing neurons. ( c ) Bar plot showing the mean E Cl in immature neurons (control, grey bar n =6; KCC2 over, black bar n =7; ** P <0.01; unpaired t -test). ( d ) Somatic KCC2 immunostaining in control and KCC2 over-expressing neuron. (Scale bar: 5 μm). ( e ) Quantification of KCC2 immunofluorescence signals in control and KCC2 transfected neurons (control, grey bar n =16; KCC2 over, black bar n =20; *** P <0.001; unpaired t -test). ( f ) Representative sIPSCs from control and KCC2 transfected neurons. ( g ) Summary of sIPSC decay kinetics in control (grey bar n =44) and KCC2 transfected neurons (black bar n =37; ** P <0.01; unpaired t -test). ( h ) Summary of sIPSC frequency in control (grey bar n =41) and KCC2 transfected neurons (black bar n =40; P >0.05; unpaired t -test). ( i ) Immunostaining of VGAT clusters (green fluorescence) in control (left panel) and KCC2 over-expressing neurons (right panel). ( j ) Summary of VGAT cluster density quantification in control (grey bar n =19) and KCC2 transfected neurons (black bar n =24; P >0.05; unpaired t -test). ( k ) Summary of tonic current amplitude in control (grey bar n =43) and KCC2 neurons (black bar n =28; * P <0.05; unpaired t -test). ( l ) Somatic immunostaining of immunofluorescence signals for α3 and α1 subunits in control and KCC2 over-expressed neurons at DIV7, scale bar 10 μm. ( m ) Quantification of immunofluorescence signals for α3 and α1 subunits at DIV7 (α3 control, grey bar n =69; KCC2 over, black bar n =75; ** P <0.01; unpaired t -test; α1 control grey bar n =104; KCC2 over black bar n =121; *** P <0.001; unpaired t -test). ( n ) Somatic immunostaining of immunofluorescence signals for δ subunit in control and KCC2 over-expressing neurons at DIV7. ( o ) Quantification of immunofluorescence signals for δ subunit (control, grey bar n =17; KCC2 over, black bar n =42; * P <0.05; unpaired t -test). Scale bar: 23 μm. Data is presented as mean±s.e.m. Full size image In the previous set of experiments, the [Cl − ] i was modified by up-regulating KCC2 protein. However, it has been shown that KCC2 is abundant at glutamatergic synapses [14] , where it acts by binding to cytoskeletal elements, to promote dendritic spine maturation [15] in a manner independent of its transporter function. To rule out the possibility that changes in sIPSC characteristics and GABA A R subunit expression result from an alteration of the structural role of KCC2, the [Cl − ] i was modified by chronically treating neurons with Bumetanide, a pharmacological agent that blocks the activity of NKCC1. Cerebellar cultures were treated for one week with Bumetanide (30 μM) starting on DIV0 ( Fig. 1b ) to replicate the timing used with KCC2 over-expression. To assess the effect of Bumetanide on the [Cl − ] i under our experimental conditions we measured E Cl in gramicidin-perforated patch in immature cultures in presence of Bumetanide. As expected, in DIV6–7 cultures, Bumetanide treatment induced a significant shift of E Cl toward more hyperpolarized values (−49.25±3.47 and −62.67±5.8 mV in control and Bumetanide, respectively; P <0.05 unpaired t -test; Fig. 3a–c ). Next, we studied the effect of chronic treatment with Bumetanide on GABAergic sIPSCs. In DIV6–7, this drug significantly accelerated the sIPSC decay kinetics ( τ mean =31.2±1.7 and 18.9±0.8 ms in control and Bumetanide, respectively; P <0.001 unpaired t -test), without affecting the sIPSC frequency ( Fig. 3d–f ). In addition, chronic Bumetanide treatment also increased the amplitude of tonic current at DIV6–7 ( Fig. 3g ). In analogy with the experiments performed with altered KCC2 expression, we next investigated the expression levels of α3−α1 and δ subunits in neurons chronically treated with Bumetanide. In DIV6–7 cultures, Bumetanide treatment reduced the expression of α3 subunit, while it increased the expression of both α1 and δ subunits with respect to control values ( Fig. 3h–k ). These immunocytochemical data are in agreement with the electrophysiological results obtained in the presence of this chloride co-transporter blocker. 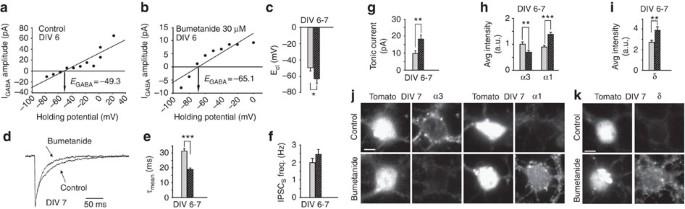Figure 3: Pharmacological treatment with Bumetanide affects GABAergic currents and regulates the expression of α3-α1 and δ subunits. (a) Example ofI–Vrelations of isoguvacine (10 μM) evoked GABAAcurrents at increasing holding potentials in control neurons. (b) Example ofI–Vrelations of isoguvacine (10 μM) evoked GABAAcurrents at increasing holding potentials in Bumetanide treated neurons. (c) Summary ofEClat DIV6–7 in control (grey barn=11) and Bumetanide treated neurons (black filled barn=13; *P<0.05; unpairedt-test). (d) Representative sIPSCs from control and Bumetanide (30 μM) treated neurons. (e) Summary of sIPSC decay kinetics in control (grey barn=26) and Bumetanide treated neurons (black filled barn=37; ***P<0.001; unpairedt-test). (f) Summary of sIPSC frequency in control (grey barn=49) and Bumetanide treated neurons (black filled barn=45;P>0.05; unpairedt-test). (g) Summary of tonic current amplitude in control (grey barn=46) and Bumetanide treated neurons (black filled barn=50; **P<0.01; unpairedt-test). (h) Quantification of immunofluorescence signals for α3 and α1 subunits (α3 control, grey barn=100; Bumetanide, black filled barn=99; **P<0.01; unpairedt-test; α1 control, grey barn=121; Bumetanide, black filled barn=119; ***P<0.001; unpairedt-test). (i) Quantification of immunofluorescence signals for δ subunit in control (grey barn=128) and in Bumetanide treated neurons (black filled barn=96; **P<0.01; unpairedt-test) at DIV6–7. (j) Somatic immunostaining of immunofluorescence signals for α3 and α1 subunits in control and Bumetanide treated neurons at DIV7. (k) Somatic immunostaining of immunofluorescence signals for δ subunit in control and Bumetanide treated neurons at DIV7. Scale bar: 23 μm. Data is presented as mean±s.e.m. Figure 3: Pharmacological treatment with Bumetanide affects GABAergic currents and regulates the expression of α3-α1 and δ subunits. ( a ) Example of I – V relations of isoguvacine (10 μM) evoked GABA A currents at increasing holding potentials in control neurons. ( b ) Example of I – V relations of isoguvacine (10 μM) evoked GABA A currents at increasing holding potentials in Bumetanide treated neurons. ( c ) Summary of E Cl at DIV6–7 in control (grey bar n =11) and Bumetanide treated neurons (black filled bar n =13; * P <0.05; unpaired t -test). ( d ) Representative sIPSCs from control and Bumetanide (30 μM) treated neurons. ( e ) Summary of sIPSC decay kinetics in control (grey bar n =26) and Bumetanide treated neurons (black filled bar n =37; *** P <0.001; unpaired t -test). ( f ) Summary of sIPSC frequency in control (grey bar n =49) and Bumetanide treated neurons (black filled bar n =45; P >0.05; unpaired t -test). ( g ) Summary of tonic current amplitude in control (grey bar n =46) and Bumetanide treated neurons (black filled bar n =50; ** P <0.01; unpaired t -test). ( h ) Quantification of immunofluorescence signals for α3 and α1 subunits (α3 control, grey bar n =100; Bumetanide, black filled bar n =99; ** P <0.01; unpaired t -test; α1 control, grey bar n =121; Bumetanide, black filled bar n =119; *** P <0.001; unpaired t -test). ( i ) Quantification of immunofluorescence signals for δ subunit in control (grey bar n =128) and in Bumetanide treated neurons (black filled bar n =96; ** P <0.01; unpaired t -test) at DIV6–7. ( j ) Somatic immunostaining of immunofluorescence signals for α3 and α1 subunits in control and Bumetanide treated neurons at DIV7. ( k ) Somatic immunostaining of immunofluorescence signals for δ subunit in control and Bumetanide treated neurons at DIV7. Scale bar: 23 μm. Data is presented as mean±s.e.m. Full size image α3-1 and δ subunits are affected by KCC2 shRNA or DIOA The effects of high [Cl − ] i on the expression of α3-α1 and δ subunits were studied in mature neurons either transfected with KCC2 shRNA or chronically treated with DIOA ( Fig. 1c,d ). Gramicidin perforated patch-clamp experiments confirmed that, at DIV12, chloride equilibrium potential ( E Cl ) was −57±2.6 mV ( Fig. 4a ), a value significantly more hyperpolarized with respect to DIV6 cultures ( Fig. 2c ). The effectiveness of KCC2 interference on the increase of [Cl − ] i on DIV12 neurons, was demonstrated by gramicidin perforated patch-clamp experiments in which the chloride equilibrium potential ( E Cl ) shifted from −57±3 to −28±1 mV ( Fig. 4a–c ). In agreement with this result, in immunocytochemistry experiments, KCC2 levels were reduced in KCC2 shRNA transfected neurons at DIV12 ( Fig. 4d,e ). Subsequently, GABAergic sIPSCs were recorded in KCC2 shRNA transfected neurons from DIV7 to DIV10–13. As previously reported, sIPSC decay kinetics accelerated during neuronal maturation [9] , [10] and, interestingly, shRNA transfection slowed down the sIPSC relaxation at any developmental stage tested, whereas it did not affect sIPSC frequency ( Fig. 4f–h ). At DIV10–13, the tonic current amplitude was also significantly decreased by KCC2 shRNA transfection ( Fig. 4i ). These electrophysiological results were corroborated by immunocytochemistry showing that KCC2 shRNA down-regulated the α1 subunit and increased the expression of the α3 subunit at DIV12 ( Fig. 4j,k ), whereas at DIV7 only a moderate decrease of α1 subunit was observed (1469.3±256.6 AU n =8; 959.6±93.3 AU n =23, for control and KCC2 shRNA, respectively; P <0.05; unpaired t -test; not shown). Furthermore, the surface expression of the δ subunit was also reduced in KCC2 shRNA transfected neurons at DIV12 ( Fig. 4l,m ). 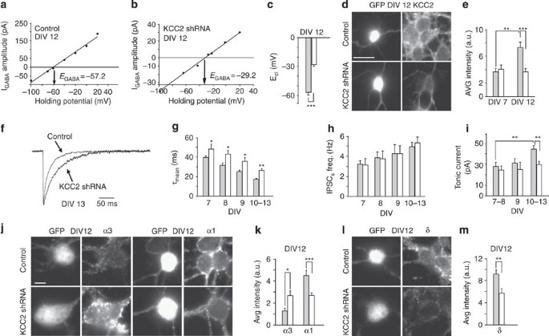Figure 4: KCC2 shRNA interference affects GABAergic currents and regulates the expression of α3-α1 and δ subunits. (a) Example ofI–Vrelations of isoguvacine (10 μM) evoked GABAAcurrents at increasing holding potentials in control neurons. (b) Example ofI–Vrelations of isoguvacine (10 μM) evoked GABAAcurrents at increasing holding potentials in KCC2 shRNA transfected neurons. (c) Summary ofEClat DIV12 in control (grey barn=15) and KCC2 shRNA transfected neurons (white barn=11; ***P<0.001; unpairedt-test). (d) Somatic KCC2 immunostaining in control and KCC2 shRNA neurons at DIV12 (Scale bar: 5 μm). (e) Quantification of KCC2 immunofluorescence signals in control and KCC2 shRNA neurons (at DIV7 control, grey barn=9; KCC2 shRNA, white barn=9;P>0.05 unpairedt-test; at DIV12 control, grey barn=12; KCC2 shRNA, white barn=12; ***P<0.001; **P<0.01; unpairedt-test). (f) Representative sIPSCs from control and KCC2 shRNA transfected neurons. (g) Summary of sIPSC decay kinetics in control (grey bar DIV7n=11; DIV8n=20; DIV9n=10; DIV10–13n=22) and KCC2 shRNA transfected neurons (white bar DIV7n=9; DIV8n=7; DIV9n=9; DIV10–13n=19; *P<0.05;**P<0.01; unpairedt-test). (h) Summary of sIPSC frequency in control (grey bar DIV7n=12; DIV8n=21; DIV9n=11; DIV10–13n=23) and KCC2 shRNA transfected neurons (white bar DIV7n=7; DIV8n=8; DIV9n=10; DIV10–13n=19;P>0.05; unpairedt-test). (i) Summary of tonic current amplitude in control (grey bar DIV7–8n=17; DIV9n=9; DIV10–13n=13) and KCC2 shRNA neurons (white bar DIV7–8n=27; DIV9n=9; DIV10–13n=25; **P<0.01; unpairedt-test). (j) Somatic immunostaining of immunofluorescence signals for α3 and α1 subunits in control and KCC2 shRNA transfected neurons at DIV12. (k) Quantification of immunofluorescence signals for α3 and α1 subunits (α3 control, grey barn=9; KCC2 shRNA, white barn=14; *P<0.5; unpairedt-test; α1 control, grey barn=15; KCC2 shRNA, white barn=21; ***P<0.001; unpairedt-test). (l) Somatic immunostaining of immunofluorescence signals for δ subunit in control and KCC2 shRNA transfected neurons. (m) Quantification of immunofluorescence signals for δ subunit in control (grey barn=20) and KCC2 shRNA expressing neurons (white barn=18; **P<0.01; unpairedt-test) at DIV12. Scale bar: 23 μm. Data is presented as mean±s.e.m. Figure 4: KCC2 shRNA interference affects GABAergic currents and regulates the expression of α3-α1 and δ subunits. ( a ) Example of I – V relations of isoguvacine (10 μM) evoked GABA A currents at increasing holding potentials in control neurons. ( b ) Example of I – V relations of isoguvacine (10 μM) evoked GABA A currents at increasing holding potentials in KCC2 shRNA transfected neurons. ( c ) Summary of E Cl at DIV12 in control (grey bar n =15) and KCC2 shRNA transfected neurons (white bar n =11; *** P <0.001; unpaired t -test). ( d ) Somatic KCC2 immunostaining in control and KCC2 shRNA neurons at DIV12 (Scale bar: 5 μm). ( e ) Quantification of KCC2 immunofluorescence signals in control and KCC2 shRNA neurons (at DIV7 control, grey bar n =9; KCC2 shRNA, white bar n =9; P >0.05 unpaired t -test; at DIV12 control, grey bar n =12; KCC2 shRNA, white bar n =12; *** P <0.001; ** P <0.01; unpaired t -test). ( f ) Representative sIPSCs from control and KCC2 shRNA transfected neurons. ( g ) Summary of sIPSC decay kinetics in control (grey bar DIV7 n =11; DIV8 n =20; DIV9 n =10; DIV10–13 n =22) and KCC2 shRNA transfected neurons (white bar DIV7 n =9; DIV8 n =7; DIV9 n =9; DIV10–13 n =19; * P <0.05;** P <0.01; unpaired t -test). ( h ) Summary of sIPSC frequency in control (grey bar DIV7 n =12; DIV8 n =21; DIV9 n =11; DIV10–13 n =23) and KCC2 shRNA transfected neurons (white bar DIV7 n =7; DIV8 n =8; DIV9 n =10; DIV10–13 n =19; P >0.05; unpaired t -test). ( i ) Summary of tonic current amplitude in control (grey bar DIV7–8 n =17; DIV9 n =9; DIV10–13 n =13) and KCC2 shRNA neurons (white bar DIV7–8 n =27; DIV9 n =9; DIV10–13 n =25; ** P <0.01; unpaired t -test). ( j ) Somatic immunostaining of immunofluorescence signals for α3 and α1 subunits in control and KCC2 shRNA transfected neurons at DIV12. ( k ) Quantification of immunofluorescence signals for α3 and α1 subunits (α3 control, grey bar n =9; KCC2 shRNA, white bar n =14; * P <0.5; unpaired t -test; α1 control, grey bar n =15; KCC2 shRNA, white bar n =21; *** P <0.001; unpaired t -test). ( l ) Somatic immunostaining of immunofluorescence signals for δ subunit in control and KCC2 shRNA transfected neurons. ( m ) Quantification of immunofluorescence signals for δ subunit in control (grey bar n =20) and KCC2 shRNA expressing neurons (white bar n =18; ** P <0.01; unpaired t -test) at DIV12. Scale bar: 23 μm. Data is presented as mean±s.e.m. Full size image In order to increase the [Cl − ] i without interfering with the expression level of the KCC2 protein, DIV5 neurons were chronically treated with the KCC2 inhibitor DIOA. Although DIOA shows only a partial specificity for KCC2 (refs 16 , 17 ) this drug caused a marked shift of E Cl in mature neurons, validating its effect in increasing [Cl − ] i (−64.96±7.5 and −45.05±8.43 mV in control and DIOA conditions, respectively; P <0.05 unpaired t -test; Fig. 5a–c ). Experiments aimed at investigating sIPSCs in the presence of DIOA showed that, in DIV12–13 cultures, this drug was able to induce a slowdown of the sIPSC current relaxation (11.8±0.8 and 24.4±1.3 ms in control and DIOA conditions, respectively; P <0.001 unpaired t -test) ( Fig. 5d,e ) and significantly decreased the sIPSC frequency ( Fig. 5f ). Chronic treatment with DIOA also decreased the tonic current at DIV12–13 ( Fig. 5g ). In addition, DIOA slightly, but significantly increased the expression of α3 subunit, while it markedly decreased the expression of both α1 and δ subunits ( Fig. 5h–k ). Also in this case, electrophysiological data paralleled the immunocytochemistry results, indicating that differences in phasic and tonic GABAergic currents under conditions of altered [Cl − ] i rely on changes in the expression of α3–α1 and δ subunits. 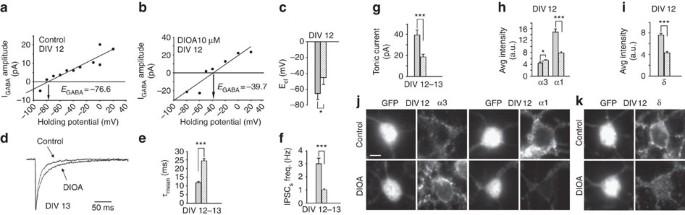Figure 5: Pharmacological treatment with DIOA affects GABAergic currents and regulates the expression of α3-α1 and δ subunits. (a) Example ofI–Vrelations of isoguvacine (10 μM) evoked GABAAcurrents at increasing holding potentials in control neurons. (b) Example ofI-Vrelations of isoguvacine (10 μM) evoked GABAAcurrents at increasing holding potentials in DIOA treated neurons. (c) Summary ofEClat DIV12 in control (grey barn=8) and DIOA treated neurons (white filled barn=8; *P<0.05; unpairedt-test). (d) Representative sIPSCs from control and DIOA (10 μM) treated neurons. (e) Summary of sIPSCs decay kinetics in control (grey barn=33) and DIOA treated neurons (white filled barn=35; ***P<0.001; unpairedt-test). (f) Summary of sIPSC frequency in control (grey barn=33) and DIOA treated neurons (white filled barn=35; ***P<0.001; unpairedt-test). (g) Summary of tonic current amplitude in control (grey barn=25) and DIOA treated neurons (white filled barn=32; ***P<0.001; unpairedt-test). (h) Quantification of immunofluorescence signals for α3 and α1 subunits (α3 control, grey barn=52; DIOA, white filled barn=55; *P<0.5; unpairedt-test; α1 control, grey barn=53; DIOA, white filled barn=59; ***P<0.001; unpairedt-test). (i) Quantification of immunofluorescence signals for δ subunit in control (grey barn=71) and DIOA treated neurons (white filled barn=41; ***P<0.001; unpairedt-test). (j) Somatic immunostaining of immunofluorescence signals for α3 and α1 subunits in control and DIOA treated neurons at DIV12. (k) Somatic immunostaining of immunofluorescence signals for δ subunit in control and DIOA treated neurons. Scale bar: 23 μm. Data is presented as mean±s.e.m. Figure 5: Pharmacological treatment with DIOA affects GABAergic currents and regulates the expression of α3-α1 and δ subunits. ( a ) Example of I – V relations of isoguvacine (10 μM) evoked GABA A currents at increasing holding potentials in control neurons. ( b ) Example of I - V relations of isoguvacine (10 μM) evoked GABA A currents at increasing holding potentials in DIOA treated neurons. ( c ) Summary of E Cl at DIV12 in control (grey bar n =8) and DIOA treated neurons (white filled bar n =8; * P <0.05; unpaired t -test). ( d ) Representative sIPSCs from control and DIOA (10 μM) treated neurons. ( e ) Summary of sIPSCs decay kinetics in control (grey bar n =33) and DIOA treated neurons (white filled bar n =35; *** P <0.001; unpaired t -test). ( f ) Summary of sIPSC frequency in control (grey bar n =33) and DIOA treated neurons (white filled bar n =35; *** P <0.001; unpaired t -test). ( g ) Summary of tonic current amplitude in control (grey bar n =25) and DIOA treated neurons (white filled bar n =32; *** P <0.001; unpaired t -test). ( h ) Quantification of immunofluorescence signals for α3 and α1 subunits (α3 control, grey bar n =52; DIOA, white filled bar n =55; * P <0.5; unpaired t -test; α1 control, grey bar n =53; DIOA, white filled bar n =59; *** P <0.001; unpaired t -test). ( i ) Quantification of immunofluorescence signals for δ subunit in control (grey bar n =71) and DIOA treated neurons (white filled bar n =41; *** P <0.001; unpaired t -test). ( j ) Somatic immunostaining of immunofluorescence signals for α3 and α1 subunits in control and DIOA treated neurons at DIV12. ( k ) Somatic immunostaining of immunofluorescence signals for δ subunit in control and DIOA treated neurons. Scale bar: 23 μm. Data is presented as mean±s.e.m. Full size image Altogether, the similar effects of KCC2 over-expression and down-regulation with respect to Bumetanide and DIOA treatments, respectively, indicate that the structural interaction of KCC2 with the cytoskeleton plays a minor role in the regulation of α3–α1 and δ subunits, and provide a first demonstration that [Cl − ] i itself is responsible for the regulation of these GABA A R subunits expression. Zolpidem and THIP revealed changes in α1 and δ subunits To further demonstrate that modulation of KCC2 protein levels affects the expression GABA A R subunits, we used a pharmacological approach exploiting Zolpidem, an allosteric modulator of GABA A Rs that when applied at low concentration preferentially enhances current mediated by α1-containing receptors [18] , [19] , and THIP, a GABA A R agonist, which selectively activates δ-containing GABA A Rs [20] . As Zolpidem has been reported to selectively prolong the decay and increase the peak amplitude of synaptic α1-containing GABA A receptors [18] , [19] , its potentiating effect on synaptic currents reflects the relative abundance of the α1 subunit in synaptic GABA A Rs. The effect of Zolpidem was studied only on the sIPSC decay kinetics, since it has been demonstrated that the amplitude enhancement exerted by this drug critically depends on the extent of postsynaptic receptor saturation [18] . Spontaneous GABAergic activity was recorded in the presence of Zolpidem (300 nM) in both DIV6–7 and DIV12–13 cultures under conditions of altered KCC2 expression. At DIV6–7, the increase of sIPSC mean decay time constant induced by Zolpidem application was significantly higher in KCC2-transfected cells with respect to control (5.0±3.5 and 18.7±6.8 ms in control and KCC2, respectively; P <0.05 ANOVA) ( Fig. 6a ). In contrast, the robust Zolpidem-induced relaxation of sIPSC decay kinetics was significantly reduced in KCC2-shRNA transfected neurons (44.6±5.9 and 17.9±4.4 ms in control and KCC2 shRNA, respectively; P <0.01 ANOVA) ( Fig. 6a ). These data suggest that the expression levels of KCC2 affect α1 subunit expression. To directly test whether up- or down-regulation of KCC2 also interferes with δ subunit expression we exogenously applied both GABA and THIP pulses and, as previously reported, the ratio between the current peak amplitude obtained in THIP and GABA ( I THIP / I GABA ) was taken as a measure of the expression of δ-containing GABA A Rs [9] , [20] . At DIV6–7, KCC2 over-expression significantly increased the I THIP / I GABA ratio (0.05±0.02 and 0.16±0.05 in control and KCC2 over, respectively; P <0.001 ANOVA), indicating an increase in δ-containing GABA A Rs with respect to control ( Fig. 6b,c ). Conversely, KCC2 shRNA reduced the I THIP / I GABA ratio (0.26±0.05 and 0.05±0.01 in control and KCC2 shRNA, respectively; P <0.001 ANOVA) indicating that KCC2 down-regulation significantly decreased the expression of extrasynaptic tonic receptors at mature stages ( Fig. 6b,d ). Taken together, these results suggest that KCC2 expression affects GABA A R subunit composition at the level of both α1 (phasic current) and δ (tonic current) subunits. 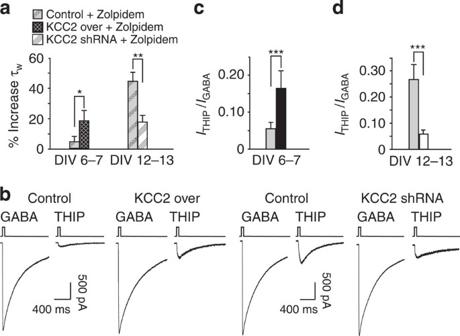Figure 6: Zolpidem and THIP reveal changes of α1-δ subunit expression in altered KCC2 expression. (a) Summary of the average percent increase in the sIPSC decay kinetics in KCC2 and KCC2 shRNA transfected neurons by application of Zolpidem (at DIV6–7 controln=6; KCC2 overn=9 *P<0.05; ANOVA; at DIV12–13 controln=9; KCC2 shRNAn=10; **P<0.01; ANOVA). (b) Representative whole-cell responses in KCC2 and KCC2 shRNA transfected neurons to applications of THIP (30 μM) and GABA (1 mM). (c) Summary of the average current densityITHIP/IGABAin KCC2 transfected neurons (control, grey barn=22; KCC2 over, black barn=22; ***P<0.001 ANOVA). (d) Summary of the average current densityITHIP/IGABAin KCC2 shRNA transfected neurons (control, grey barn=12; KCC2 shRNA, white barn=12; ***P<0.001 ANOVA). Data is presented as mean±s.e.m. Figure 6: Zolpidem and THIP reveal changes of α1-δ subunit expression in altered KCC2 expression. ( a ) Summary of the average percent increase in the sIPSC decay kinetics in KCC2 and KCC2 shRNA transfected neurons by application of Zolpidem (at DIV6–7 control n =6; KCC2 over n =9 * P <0.05; ANOVA; at DIV12–13 control n =9; KCC2 shRNA n =10; ** P <0.01; ANOVA). ( b ) Representative whole-cell responses in KCC2 and KCC2 shRNA transfected neurons to applications of THIP (30 μM) and GABA (1 mM). ( c ) Summary of the average current density I THIP / I GABA in KCC2 transfected neurons (control, grey bar n =22; KCC2 over, black bar n =22; *** P <0.001 ANOVA). ( d ) Summary of the average current density I THIP / I GABA in KCC2 shRNA transfected neurons (control, grey bar n =12; KCC2 shRNA, white bar n =12; *** P <0.001 ANOVA). Data is presented as mean±s.e.m. Full size image Chloride ions affect α3−1 and δ subunits expression Early GABAergic signaling triggers elevation in the intracellular Ca 2+ concentration which plays an important trophic role for developing networks [6] , [12] . To rule out the possibility that the changes in GABA A R subunits expression induced by KCC2 over-expression or down-regulation are due to trophic alterations resulting from the lack or persistence of GABAergic depolarization during neuronal development, we investigated the kinetics of GABAergic synaptic currents in neurons with altered KCC2 expression which were chronically treated with the non-competitive GABA A R antagonist picrotoxin (PTX). Similar to the data reported in Figs 2g and 4g , KCC2 over-expressing neurons chronically treated with PTX showed faster sIPSC decay kinetics (40.41±4.7 and 29.23±1.65 ms in control and KCC2 over-expression, respectively; P <0.01 unpaired t -test; Fig. 7a,c ) whereas neurons expressing KCC2 shRNA displayed slower sIPSC decay kinetics (26.56±2.3 and 35.13±3.19 in control and KCC2 shRNA, respectively; P <0.05 unpaired t -test; Fig. 7b,c ). These observations suggest that the effect exerted by [Cl − ] i on the α3-α1 and δ GABA A R subunit expression does not depend on the trophic support provided by GABAergic signaling. 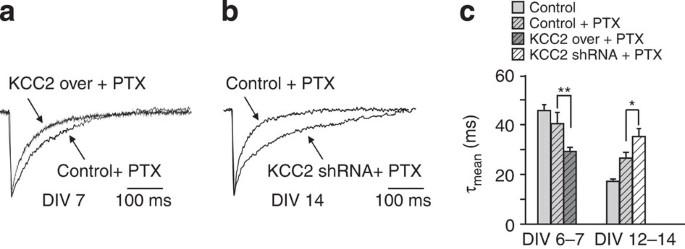Figure 7: Picrotoxin chronic treatment does not prevent the effects exerted by altered KCC2 expression on sIPSCs kinetics. (a) Representative sIPSCs traces from control and KCC2 over-expressing neurons chronically treated with PTX at DIV7. (b) Representative sIPSCs traces from control and KCC2 shRNA transfected neurons chronically treated with PTX at DIV14. (c) Summary of sIPSC decay kinetics in KCC2 and KCC2 shRNA transfected neurons chronically treated with 100 μM PTX (at DIV6–7 controln=44; PTX controln=9; PTX KCC2 overn=17; **P<0.01; at DIV12–13 controln=22; PTX controln=7; PTX KCC2 shRNAn=12; *P<0.05; unpairedt-test). Data is presented as mean±s.e.m. Figure 7: Picrotoxin chronic treatment does not prevent the effects exerted by altered KCC2 expression on sIPSCs kinetics. ( a ) Representative sIPSCs traces from control and KCC2 over-expressing neurons chronically treated with PTX at DIV7. ( b ) Representative sIPSCs traces from control and KCC2 shRNA transfected neurons chronically treated with PTX at DIV14. ( c ) Summary of sIPSC decay kinetics in KCC2 and KCC2 shRNA transfected neurons chronically treated with 100 μM PTX (at DIV6–7 control n =44; PTX control n =9; PTX KCC2 over n =17; ** P <0.01; at DIV12–13 control n =22; PTX control n =7; PTX KCC2 shRNA n =12; * P <0.05; unpaired t -test). Data is presented as mean±s.e.m. Full size image To further investigate the causal link between changes in [Cl − ] i variations and expression of distinct α subunits, KCC2 was down-regulated in mature neurons (DIV12) ( Fig. 1e ), when both the shift in the polarity of chloride gradient and the α3 to α1 switch had already occurred and examined α subunit expression and IPSCs characteristics under these conditions. As shown in Fig. 8a,b , sIPSCs recorded from DIV14 neurons transfected with KCC2 shRNA at DIV12, showed significantly slower decay kinetics with respect to control (18.9±1.1 and 28.1±2.5 ms in control and KCC2 shRNA, respectively; P <0.01 unpaired t -test). In line with this observation, immunocytochemistry experiments showed that KCC2 shRNA transfection up-regulated the α3 subunit, whereas it considerably reduced α1 subunit expression ( Fig. 8d,e ). In addition, neurons with down-regulated levels of KCC2 showed smaller tonic currents ( Fig. 8c ), an observation corroborated by the lower δ immunoreactivity in KCC2 shRNA neurons ( Fig. 8d,f ). Taken together, these data suggest that the α3 to α1 subunit switch and the expression of δ subunit strictly correlate with [Cl − ] i, whereas they are independent of the trophic effect of depolarizing GABA and of the stages of neuronal development. 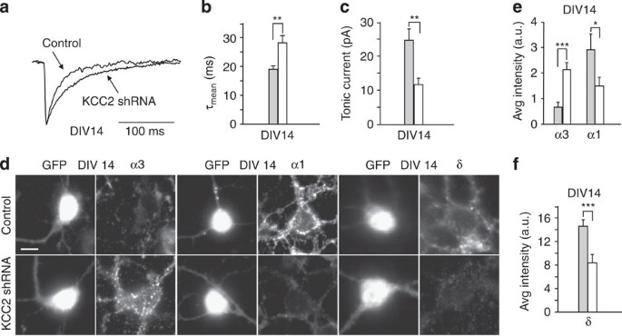Figure 8: Transfection of KCC2 shRNA at mature developmental stage affects the α3-α1 and δ subunit expression. (a) Representative sIPSCs traces in control and KCC2 shRNA transfected neurons at DIV14. (b) Summary of sIPSC decay kinetics in control and KCC2 shRNA transfected neurons (control, grey barn=18; KCC2 shRNA, white barn=25; **P<0.01; unpairedt-test). (c) Summary of tonic currents in control and KCC2 shRNA transfected neurons (control, grey barn=10; KCC2 shRNA, white barn=24; **P<0.01; unpairedt-test). (d) Representative somatic immunostaining of α3, α1 and δ subunits in control and KCC2 shRNA transfected neurons. (e) Quantification of immunofluorescence signals for α3 and α1 subunits (α3 control, grey barn=16; KCC2 shRNA, white barn=23; ***P<0.001; unpairedt-test; α1 control, grey barn=16; KCC2 shRNA, white barn=12; *P<0.05; unpairedt-test). (f) Quantification of immunofluorescence signals for δ subunit (control, grey barn=34; KCC2 shRNA, white barn=16; ***P<0.001; unpairedt-test). Scale bar: 23 μm. Data is presented as mean±s.e.m. Figure 8: Transfection of KCC2 shRNA at mature developmental stage affects the α3-α1 and δ subunit expression. ( a ) Representative sIPSCs traces in control and KCC2 shRNA transfected neurons at DIV14. ( b ) Summary of sIPSC decay kinetics in control and KCC2 shRNA transfected neurons (control, grey bar n =18; KCC2 shRNA, white bar n =25; ** P <0.01; unpaired t -test). ( c ) Summary of tonic currents in control and KCC2 shRNA transfected neurons (control, grey bar n =10; KCC2 shRNA, white bar n =24; ** P <0.01; unpaired t -test). ( d ) Representative somatic immunostaining of α3, α1 and δ subunits in control and KCC2 shRNA transfected neurons. ( e ) Quantification of immunofluorescence signals for α3 and α1 subunits (α3 control, grey bar n =16; KCC2 shRNA, white bar n =23; *** P <0.001; unpaired t -test; α1 control, grey bar n =16; KCC2 shRNA, white bar n =12; * P <0.05; unpaired t -test). ( f ) Quantification of immunofluorescence signals for δ subunit (control, grey bar n =34; KCC2 shRNA, white bar n =16; *** P <0.001; unpaired t -test). Scale bar: 23 μm. Data is presented as mean±s.e.m. Full size image Our findings provide evidence for a physiological role of neuronal [Cl − ] i , in regulating the expression of various GABA A R subtypes, thereby tuning phasic and tonic GABAergic inhibition independently of GABAergic signaling. It has been recently demonstrated that intracellular chloride ions bind to specific sites in the GABA A R pore affecting the receptor gating [21] , [22] . Our observations further extend the hypothesis that [Cl − ] i acts as a intracellular messenger exerting a feedback control on GABA A currents not only by interfering with GABA A R gating, but also by modulating the expression of GABA A R subunits. The latter mechanism would therefore represent an additional level of complexity in the role of neuronal chloride homeostasis. A growing body of evidence indicates that chloride is unevenly distributed across neuronal sub-compartments, although this issue is still a matter of debate and its physiological relevance has not been fully elucidated [23] , [24] , [25] , [26] , [27] , [16] . Along this line, it has been recently proposed that, in the hippocampus, chloride homeostasis can be regulated at the level of individual synapses [28] . Indeed, perisomatic inhibitory synapses formed between parvalbumin positive (PV + ) interneurons and CA1 hippocampal pyramidal neurons are selectively modulated by ClC-2, a channel which extrudes excess of chloride under conditions of sustained activity. In contrast, CCK + interneuron synapses onto CA1 pyramidal neurons, also located in the somatic region of CA1 pyramidal neurons, do not show this [Cl − ] i regulation. Interestingly, synapses formed by PV + interneuron onto CA1 pyramidal neurons express α1-containing GABA A Rs, whereas CCK + interneuron-CA1 synapses express α2-containing GABA A Rs [29] . Although the actual occurrence of chloride micro-domains is still a matter of debate, it is tempting to speculate that GABA A R subtypes composition could be regulated by [Cl − ] i in a synaptic-specific fashion. In the present study, we found that over-expression of KCC2 does not affect the frequency of sIPSCs. These findings appear counterintuitive, since the early GABA depolarizing action has been shown to promote the morphological maturation of the neurons [30] . Nevertheless, the effect of [Cl − ] i reduction at early developmental stage on the frequency of spontaneous GABAergic synaptic currents observed in previous studies, is controversial [31] , [32] , [33] , [34] . This discrepancy could depend on the various approaches used to decrease the [Cl − ] i such as KCC2 over-expression, NKCC1 shRNA or Bumetanide treatment. In addition further variability could be due to the different developmental stage at which [Cl − ] i manipulation is performed and the neuronal type analyzed. The same considerations could be invoked to explain the discrepancy between our results and previous investigations on the sIPSC frequency in chronic treatment with DIOA [35] . The chronic pharmacological blockade of GABA A Rs during development has been shown to produce a significant delay of the [Cl − ] i shift [36] . This observation is in agreement with our results showing that chronic treatment with picrotoxin (PTX) induced slower sIPSC decay kinetics in DIV12–14 neurons ( Fig. 7c ), supporting the notion that [Cl − ] i regulates GABAergic PSC decay kinetics and α subunits expression. We observe that the E Cl in shRNA KCC2 neurons was considerably shifted toward positive values ( Fig. 4c ). This could be explained by a residual expression of NKCC1 (refs 16 , 37 ) and/or by other yet unidentified chloride uptake mechanisms. Our data emphasize the role of [Cl − ] i in regulating the α3-α1 and δ subunit expression and therefore the decay kinetics of GABAergic PSCs and the tonic inhibition. At this stage, however, it is not clear whether the dependence of α3-α1 and δ subunit expression on [Cl − ] i is due to alteration of transcription, translation, trafficking, targeting or post-transcriptional modifications of such GABA A R subunits. In these various scenarios, chloride ions would exert their effects either by binding directly to GABA A Rs and/or by acting through GABA A R subunit-interacting-proteins or transcription factors. In addition, altered [Cl − ] i could interfere with other mechanisms including intracellular pH (ref. 38 ) or glutamate reuptake [39] . It has been reported that KCC2 structurally associates with the cytoskeleton and participates in controlling spine morphology, an effect that does not involve its ionic transport function [15] . KCC2 down-regulation, therefore, would interfere with glutamatergic function which, in turn, may alter GABAergic transmission. Although this is a plausible possibility, our experiments show that modifying [Cl − ] i without interfering with the KCC2 expression level, exerts a similar effect on α3-α1 and δ expression with respect to KCC2 over-expression and down-regulation. The majority of neurons analyzed in the present study have been classified as stellate/basket cells, based on their morphology and immunoreactivity to specific interneuronal markers (Methods). Although most of the studies characterizing the α3/α1 and δ subunits switch have been carried out in granule cells, we show here that, in stellate/basket cells in culture, the developmental expression of such subunits appears to be comparable to that observed in granule cells. Those findings are confirmed by works in both cerebellar stellate/basket interneurons and hippocampal PV + interneurons showing a developmental increase of α1-containing receptors associated with increases in KCC2 levels [40] , [41] . In keeping with this, our model is validated by the fact that, in our experiments, the developmental chloride inversion occurs at the same time of α3/α1 subunit switch and δ subunit increase. Under physiological conditions of sustained hyperpolarizing GABAergic activity, accumulation of [Cl − ] i would induce smaller IPSC peak amplitude by lowering the driving force of the chloride current. It can be speculated that, in these scenario, slower GABAergic currents would homeostatically regulate the amount of GABAergic charge transfer by prolonging the IPSC duration. Conversely, under pathologic conditions, in which the increase of [Cl − ] i may lead to depolarizing actions [42] , [43] , [44] , the IPSCs slow-down together with the lower shunting inhibition due to the reduced tonic GABA A conductance could contribute in determining an enhancement of the aberrant excitatory GABA action. CGC cell culture and chronic treatment All the experiments involving mice were performed in accordance with Italian Ministry of Health. Primary cultures of cerebellar granule cells (CGCs) were prepared from cerebella of postnatal day 7 mice. After decapitation of the pups, we collected cerebella and subsequently we removed the meninges, as well as any large blood vessels or extraneous brain regions that are stuck to the cerebella. We chopped the tissue finely in 2 directions and then we centrifuge at 1,000 r.p.m. for 2 min. Tissue were dissociated with 0.25 mg/ml trypsin (Invitrogen, Italy) for 15 min at 37 °C in water bath and gently swirl the cerebella every 5 min. After dissociation of the cells, CGCs were plated in 12 well dishes at a density of 1×10 6 cells/ml on glass coverslips coated with poly- D -lysine (0.1 μg/ml) (Sigma, Italy). Cells were cultured in basal Eagle's medium supplemented with 10% fetal bovine serum, 2 mM glutamine, and 100 μg/ml gentamycin (Invitrogen, Italy) and maintained at 37 °C in 5% CO 2 . The final concentration of KCl in the culture medium was adjusted to 25 mM (high K + ). Four days after plating, to achieve functional synapse formation, the medium was replaced with low (5 mM) K + medium (MEM, Invitrogen, Italy) supplemented with 5 mg/ml glucose, 0.1 mg/ml transferrin, 0.025 mg/ml insulin, 2 mM glutamine, 20 μg/ml gentamicin. 5 μM cytosine arabinofuranoside (Sigma, Italy) was added to all cultures to inhibit glial proliferation. Control (pRNAT-U6.3-cGFP) and KCC2 RNA interference (KCC2 shRNA) vectors were transfected into neurons at 5 days in vitro (DIV5) or DIV12 using Effectene reagent according to the manufacturer's recommendations (Qiagen, Valencia, CA, USA). Nucleofection of CGCs with control (pCAG-IRES-tdTomato) and KCC2 over-expressing (pCAG-KCC2IRES-tdTomato) [30] was performed at DIV0 following the manufacturer's protocol (Amaxa, Gaithersburg, MD). CGCs cultures represent a mixed neuronal population mainly composed by granule cells and stellate/basket interneurons. In the attempt to assess whether transfection occurred preferentially in one of these two neuronal subtypes, we studied the soma area of the GFP- or td-Tomato-transfected neurons as the size of granule cells is markedly smaller than that of stellate/basket interneurons. The distribution of the soma diameter of transfected cells was clearly bimodal and peaked at ~8 and 12 μm. Interestingly, the distribution of non-transfected cells corresponded to the lower peak of the aforementioned distribution. The cell size relative to the peaks of the bimodal distribution was similar to the values reported for granule cells and stellate/basket cell, respectively [9] , [45] . The formal fit of the bimodal distribution indicated that the relative component of granule cells versus interneurons was ~0.3. Immunocytochemistry experiments where GABAergic interneurons were stained with anti-GAD65 antibody confirmed this estimation (data not shown). This suggests that interneurons represented the major population of GFP- or td-Tomato-transfected neurons. Chronic treatments with PTX (100 μM, Sigma, Italy) and R-(+)-[(dihydroindenyl)oxy] (DIOA) (10 μM, Sigma, Italy) were started at DIV5 in control and in KCC2 shRNA transfected neurons. The same treatment with PTX and Bumetanide (30 μM, Sigma, Italy) were started the day of plating (DIV0) in control and KCC2 over-expressing neurons. Plasmid constructs A small hairpin RNA plasmid interfering with the expression of KCC2 (KCC2 shRNA), was designed using the GenScript target finder. Two complementary annealed oligonucleotides (Top oligo 5′-GGATCCCGTAAGTGGTACAGAAACGTGGTTTGATATCCGACCACGTTTCTGTACCACTTATTTTTTCCAAA-3′; Bottom oligo 5′-AAGCTTTTGGAAAAAATAAGTGGTACAGAAACGTGGTCGGATATCAAACCACGTTTCTGTACCACTTACGG-3′) targeting a 21-nucleotide stretch in KCC2 were inserted between the BamHI and HindIII sites of the pRNAT-U6.3-cGFP vector (GenScript) to generate the KCC2 shRNA construct. A non-silencing control shRNA vector was engineered identically, except that the KCC2 target sequence was substituted by a 21-nucleotides sequence (5′-AATTCTCCGAACGTGTCACGT-3′) bearing no significant homology to any mammalian gene. The identity of both shRNA constructs were verified by sequencing. Immunocytochemistry and epifluorescence microscopy Surface live immunolabeling of α1, α3 and δ subunits was performed by incubating cultured neurons with the appropriate antibody for 10 min (α1—1:300 and α3—1:200) (Alomone, Israel) (δ—1:100) (a gift of Professor W. Sieghart, Medical University of Vienna, Austria). After washing in phosphate-buffered saline (PBS) (Invitrogen, Italy), neurons were fixed in 4% paraformaldehyde - 4% sucrose and then blocked in PBS containing 10% horse serum and 0.5% bovine serum albumin. For immunostaining of KCC2, VGAT and GAD65 cells were permeabilized with 0.1% Triton X-100 for 10 min in blocking solution and incubated with anti-KCC2 primary antibody (1:100, Millipore), VGAT primary antibody (1:400, Synaptic Systems, Germany) or GAD65 primary antibody (1:100) for 1 h at room temperature. Alexa568- and Alexa488-conjugated anti-rabbit secondary antibodies (Molecular Probes, Invitrogen, Italy) were used at 1:500 and incubated for 30 min at room temperature. Coverslips were mounted in DAKO fluorescence mounting medium and observed using a 60× objective (1.4 NA) on a wide field inverted fluorescence microscope (Nikon Eclipse Ti). Samples were illuminated with a mercury lamp and appropriate filter cubes (Semrock, Italy) for Alexa568 and Alexa488 fluorescence. Images were acquired with a digital camera (Hamamatsu EM-CCD C9100) using MetaMorph 7.5 (Molecular Devices). The same software was also used for quantitative analysis of acquired images. The analysis was restricted to the soma of transfected neurons identified by fluorescence-tagged recombinant proteins (EGFP or td-Tomato). Receptor quantity was calculated as the integrated fluorescence intensity measured on the soma, divided by its area. Background fluorescence was subtracted from all images before analysis. Control experiments without the primary antibodies were performed to test fluorescence signal arising from non specific binding of secondary antibodies. Electrophysiology recordings Spontaneous inhibitory postsynaptic currents (sIPSCs) were recorded from 6 to 14 DIV neurons in the whole-cell voltage clamp configuration at room temperature and holding potential of −60 mV, using the 700B Axopatch amplifier (Molecular Devices, Sunnyvale, CA). Patch pipettes were pulled from borosilicate glass capillaries and displayed resistance ~5–10 MΩ when filled with high chloride intracellular solution containing (in mM): 122 CsCl; 2 MgCl 2 ; 2 CaCl 2 ; 4 Na 2 ATP; 11 BAPTA; 10 HEPES; (300 mOsm and pH 7.2). Extracellular solution contained (in mM): 145 NaCl, 2 KCl, 2 MgCl 2 , 2 CaCl 2 , 10 HEPES, 10 glucose, and 10 μM D -serine, adjusted to pH 7.4 with NaOH. sIPSCs detection was performed using the sliding template method of the Clampfit 10.1 software (Molecular Devices, Sunnyvale, CA). Traces were acquired at 50 KHz, filtered off-line at 1 KHz using the Clampfit Bessel digital filter. On the average, three hundred events were collected for each recorded cell. Double events were rejected from analysis of kinetics and amplitude. Events were aligned at 20% of the 10–90% rise time and the current decay was fitted according to the function: y ( t )=Σ A i exp(− t/τ i ), where Ai are the fractions of respective components (Σ A i =1) and τ i are the time constants. The weighted deactivation time constant was calculated using the formula τ w =Σ τ i Ai . Gramicidin perforated patch experiments were used to measure the chloride equilibrium potential ( E Cl ). Intracellular solution contained (in mM): 150 KCl; 2 MgCl 2 ; 2 CaCl 2 ; 4 Na 2 ATP; 11 BAPTA; 10 HEPES (300 mOsm and pH 7.2). Gramicidin was added to the intracellular solution at a final concentration of 80 μg/ml from a stock 10 mg/ml in DMSO. The tip of the patch pipette was filled with normal intracellular solution, while the rest of the pipette contained the gramicidin-containing solution. Currents were evoked by puff-applying isoguvacine (10 μM) to the neuron soma through a micropipette coupled to an electrically gated pressure valve (Picospritzer III, Parker, Cleveland, OH, USA) at pulse duration of 50 ms and pressure 20 kPa. The holding potential was increased at 10 mV steps. E Cl − was determined as the x -axis intercepts point of the resulting I – V curve. Tonic current amplitudes were measured as the baseline-shift induced by the bath application of the GABA A R antagonist bicuculline methobromide (10 μM). The values of baseline current in control and in bicuculline were calculated by Gaussian fit of the component relative to the white noise of the all-point histogram relative to 5–10 s trace portions [46] . Only recordings exhibiting stable baseline were included in the analysis. GABA (application of a saturating concentration at 1 mM to estimate the total function of GABA A Rs) and 4,5,6,7-tetrahydroisoxazolo[5,4-c]pyridin-3-ol (THIP) (30 μM) were prepared in water and diluted to the desired concentration in extracellular solution. Both drugs were locally applied through Picospritzer as above. The ratio of THIP to GABA was calculated as the average of THIP current densities normalized to the average of currents densities elicited by GABA. Zolpidem, (a gift of Professor G. Bonanno, University of Genoa, Italy) a preferential modulator of α1-contaning GABA A Rs, was dissolved in water in stock solution (3 mM) and diluted to the concentration of 300 nM in extracellular solution for bath application. Statistical analysis Values are expressed as means±s.e.m. (standard error of the mean) throughout. Unless otherwise stated, statistical analysis was performed using the paired or unpaired Student's t -tests to compare two experimental groups and ANOVA followed by the Tukey's multiple comparison test when more than two experimental groups were analyzed. Statistical significance was abbreviated as follows: * P <0.05, ** P <0.01, *** P <0.001. How to cite this article: Succol, F. et al . Intracellular chloride concentration influences the GABA A receptor subunit composition. Nat. Commun. 3:738 doi: 10.1038/ncomms1744 (2012).